Visualization of a polytopic membrane protein during SecY-mediated membrane insertion The biogenesis of polytopic membrane proteins occurs co-translationally on ribosomes that are tightly bound to a membrane-embedded protein-conducting channel: the Sec-complex. The path that is followed by nascent proteins inside the ribosome and the Sec-complex is relatively well established; however, it is not clear what the fate of the N-terminal transmembrane domains (TMDs) of polytopic membrane proteins is when the C-terminal TMDs domains are not yet synthesized. Here, we present the sub-nanometer cryo-electron microscopy structure of an in vivo generated ribosome-SecY complex that carries a membrane insertion intermediate of proteorhodopsin (PR). The structure reveals a pre-opened Sec-complex and the first two TMDs of PR already outside the SecY complex directly in front of its proposed lateral gate. Thus, our structure is in agreement with positioning of N-terminal TMDs at the periphery of SecY, and in addition, it provides clues for the molecular mechanism underlying membrane protein topogenesis. Most α-helical integral membrane proteins (IMPs) enter their target membrane co-translationally via the canonical protein-conducting channel (PCC), the Sec-complex: Sec61αβγ in the ER membrane of eukaryotes; SecYEG in the cytoplasmic membrane of prokaryotes [1] . To this end, the translating ribosome is targeted to the membrane by the signal recognition particle where it binds to the Sec-complex. It has been suggested that hydrophobic transmembrane domains (TMDs) of nascent IMPs egress from the Sec-complex via a so-called lateral gate region in SecY/Sec61α between helices 2b and 7. However, evidence for the usage of the gate by polytopic IMPs is indirect, that is, crosslinking studies with a secretory protein [2] and crystal structures of laterally opening non-translocating Sec-complexes [3] , [4] , [5] , [6] . Structural evidence is limited to monotopic IMPs [7] , [8] that represent only a minor fraction of membrane proteomes. The correct topology of IMPs is determined during membrane insertion and follows the so-called positive inside rule [9] , which states that intracellular TMD-flanking loop regions carry overall more net positive charge than extracellular loop regions. Yet, the distribution of charged residues in the IMP is not the only determinant for membrane topology [10] , the Sec-complex itself [11] , [12] and the lipid composition of the membrane [13] also have determining roles. On a molecular level, however, the mechanism of membrane topogenesis remains poorly understood. Here, we visualize a nascent polytopic IMP during SecY-mediated membrane insertion, which provides novel insights into (i) the requirements for tight binding of the ribosome to SecY; (ii) interactions of a nascent IMP with SecY during biogenesis; and (iii) the retention of positively charged residues of IMPs on the cytoplasmic side of the membrane. Purification of in vivo assembled RNCs With the aim to visualize nascent IMPs during Sec-mediated membrane insertion, we first established a procedure to purify sufficient amounts of uniformly stalled stable ribosome nascent-chain complexes (RNCs) from whole Escherichia coli cells ( Fig. 1 ). The advantages of in vivo over in vitro RNC purifications are several-fold: The RNCs are generated under entirely physiological conditions and the purifications are faster, cheaper and can be easily scaled up. We used the efficient tryptophan-dependent stalling sequence of TnaC [14] in combination with an E. coli strain with artificially high intracellular tryptophan levels [15] that lacks the tmRNA system [14] . This protocol allows ~100 pmol of RNCs with a homogeneous peptidyl-tRNA to be routinely obtained from 1 liter of culture medium. 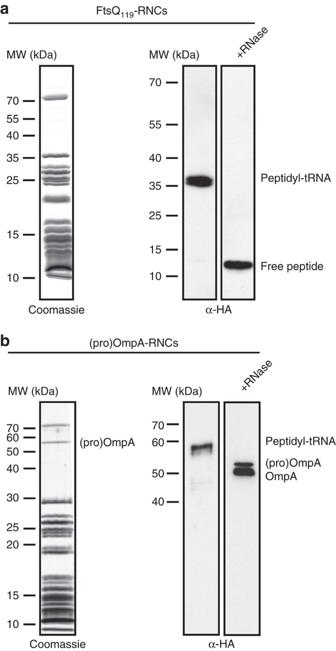Figure 1: Purification ofin vivoassembled ribosome nascent chain complexes. RNCs were purified via N-terminal affinity tags (Supplementary Figure 1andSupplementary Table 1) (a) Coomassie stained SDS–polyacrylamide gel electrophoresis gel of the ribosome nascent chain complexes of FtsQ119-RNCs and (pro-)OmpA-RNCs, showing nascent chain-tRNA of (pro-)OmpA as an extra band among the ribosomal proteins. FtsQ119-tRNA is not visible as it is hidden behind ribosomal proteins. (b) Western blot analysis of FtsQ119-RNCs and (pro-)OmpA-RNCs showing a single band for the peptidyl-tRNA that was verified by incubation of the RNCs with RNase. Figure 1: Purification of in vivo assembled ribosome nascent chain complexes. RNCs were purified via N-terminal affinity tags ( Supplementary Figure 1 and Supplementary Table 1 ) ( a ) Coomassie stained SDS–polyacrylamide gel electrophoresis gel of the ribosome nascent chain complexes of FtsQ 119 -RNCs and (pro-)OmpA-RNCs, showing nascent chain-tRNA of (pro-)OmpA as an extra band among the ribosomal proteins. FtsQ 119 -tRNA is not visible as it is hidden behind ribosomal proteins. ( b ) Western blot analysis of FtsQ 119 -RNCs and (pro-)OmpA-RNCs showing a single band for the peptidyl-tRNA that was verified by incubation of the RNCs with RNase. Full size image Requirements for tightly-coupled RNC-SecY complexes Next, we sought for mild conditions under which the SecY complex could be co-purified with RNCs of two model IMPs: the well-characterized monotopic (type II) IMP FtsQ [16] , and the polytopic IMP proteorhodopsin (PR) [17] . The latter was chosen because (i) it has a relatively simple membrane topology of seven TMDs connected by short hydrophilic loops, (ii) its three-dimensional structure is known [18] and (iii) an affinity tag placed directly after the signal sequence cleavage site [17] in the periplasm is likely to be accessible for affinity purification without interfering with membrane insertion. RNC-SecY complexes were purified via the N-terminal affinity tag in the nascent chains. Although modest amounts of the SecY complex could already be co-purified with the shorter FtsQ 85 construct, more efficient co-purification of SecY was observed with the longer FtsQ 119 construct that is expected to form a hairpin structure in the PCC [19] ( Fig. 2a ). Surprisingly, however, SecY was not co-purified with any of the RNCs derived from truncated PR generated via translational stalling in any of the hydrophilic loop regions ( Fig. 2a and Supplementary Fig. 1 ). This observation suggests that the SecY-ribosome interaction can alternate between a stable (tight) and a less robust (loose) coupling. Given that hydrophobic TMDs rapidly leave the Sec-complex [20] , [21] , we tested whether a hydrophilic stretch directly following a type II TMD, as present in FtsQ 119 , may be required for tight coupling and efficient co-purification of SecY. Indeed, when RNCs carrying the first two, four or six TMDs of PR were augmented with the hydrophilic stretch of FtsQ (termed PRxQs), SecY was co-purified in amounts comparable with FtsQ 119 ( Fig. 2a ). To exclude that these chimeric model proteins artificially induce tight coupling, we also analysed the well-studied SecY substrate CyoA [22] , which has an equivalent pattern of hydrophobic TMDs and hydrophilic loops as PR2Q. Indeed, with CyoA RNCs, we could co-purify a similar amount of SecY as with our PRxQ model proteins ( Fig. 2a ). On the other hand, SecY was only loosely coupled and did not co-purify with (i) RNCs of FtsQ 119 where the hydrophilic stretch was replaced with a TMD from PR, (ii) RNCs of a posttranslational SecY substrate (pro-)OmpA and (iii) RNCs of (pro-)OmpA augmented with the hydrophilic stretch of FtsQ ( Fig. 2b ). Finally, binding behaviour changes from tightly coupled to loosely coupled upon elongation of the hydrophilic FtsQ stretch by more than 25 amino acids, resulting in less efficient SecY co-purification ( Fig. 2c ). Taken together, these findings suggest that for a tight interaction between SecY and the ribosome it is necessary that (i) the mode of translocation is co-translational and that (ii) at least one TMD with type II topology is directly followed by a hydrophilic region of not more than 90–95 amino acids length. Notably, on this basis we generated under native conditions tightly coupled ribosome-Sec complexes carrying nascent IMPs and purified them for structural studies by cryo-electron microscopy (cryo-EM). 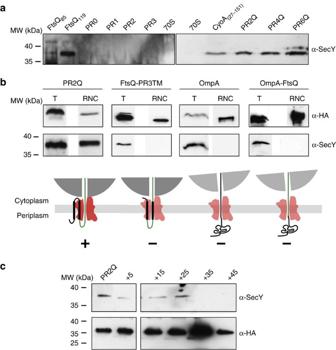Figure 2: Purification of tightly coupled RNC-SecY complexes. All RNCs were purified via an N-terminal Twin-Strep affinity tag on the nascent chain (Supplementary Figure 1b). T, sample taken from the total cleared cell lysate; RNC, sample taken from the final RNC sample. (a) Western blot analysis for co-purified SecY with RNCs derived from FtsQ, PR and CyoA. (b) Tight coupling of RNC-SecY complexes requires a co-translational mode of translocation and a hydrophilic stretch following a hydrophobic TMD. Below: schematic illustration of tightly coupled (+) and loosely (−) coupled RNC-SecY complexes. (c) Elongation of the hydrophilic stretch of PR2Q by 25 amino acids converts the RNC-SecY complex from tightly coupled to loosely coupled. Figure 2: Purification of tightly coupled RNC-SecY complexes. All RNCs were purified via an N-terminal Twin-Strep affinity tag on the nascent chain ( Supplementary Figure 1b ). T, sample taken from the total cleared cell lysate; RNC, sample taken from the final RNC sample. ( a ) Western blot analysis for co-purified SecY with RNCs derived from FtsQ, PR and CyoA. ( b ) Tight coupling of RNC-SecY complexes requires a co-translational mode of translocation and a hydrophilic stretch following a hydrophobic TMD. Below: schematic illustration of tightly coupled (+) and loosely (−) coupled RNC-SecY complexes. ( c ) Elongation of the hydrophilic stretch of PR2Q by 25 amino acids converts the RNC-SecY complex from tightly coupled to loosely coupled. Full size image Structure of a tightly-coupled RNC-SecY complex We co-purified RNCs carrying the two first TMDs from PR followed by the FtsQ hydrophilic loop with C-terminally His-tagged SecY ( Supplementary Fig. 2 ) and subjected them to cryo-EM and single particle analysis according to standard procedures. Application of several global [23] , [24] and focused [25] sorting schemes of the data set in silico resulted in a stable subpopulation of 47,471 particles that could be refined to an overall resolution of 7.3 Å according to the FSC 0.5 criterion ( Supplementary Fig. 3a ). The overall appearance of the structure is a programmed 70S ribosome with an additional density at the ribosomal exit tunnel accounting for a monomeric SecY complex, in which several rod-like elements can be observed ( Fig. 3a–c ). 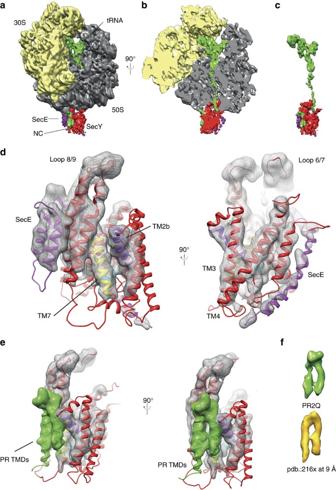Figure 3: Cryo-EM reconstruction of a tightly coupled RNC-SecY complex. (a) Overall cryo-EM structure of RNCs of PR2Q with co-purified SecY at 7.3 Å. The 30S ribosomal subunit is depicted in yellow, the 50S subunit in grey, SecY in red, SecE in magenta and the nascent chain PR2Q in green. (b) Electron density cut perpendicular to the membrane, visualizing the nascent chain in the ribosomal exit tunnel, the nascent chain can be traced from the PTC through the whole ribosomal exit tunnel. Inside SecY the nascent could not be visualized. (c) Isolated electron density for P-site tRNA; the nascent chain PR2Q and SecYE. (d) Homology model ofE. coliSecYE fitted into the isolated electron density after manual adjustment of helices. (e) Positioning of TMDs 1 and 2 of PR directly in front of the lateral gate of SecY. (f) Isolated electron density assigned to the TMDs from PR (up) displays high similarity to the corresponding domains in the NMR structure (down)18. Figure 3: Cryo-EM reconstruction of a tightly coupled RNC-SecY complex. ( a ) Overall cryo-EM structure of RNCs of PR2Q with co-purified SecY at 7.3 Å. The 30S ribosomal subunit is depicted in yellow, the 50S subunit in grey, SecY in red, SecE in magenta and the nascent chain PR2Q in green. ( b ) Electron density cut perpendicular to the membrane, visualizing the nascent chain in the ribosomal exit tunnel, the nascent chain can be traced from the PTC through the whole ribosomal exit tunnel. Inside SecY the nascent could not be visualized. ( c ) Isolated electron density for P-site tRNA; the nascent chain PR2Q and SecYE. ( d ) Homology model of E. coli SecYE fitted into the isolated electron density after manual adjustment of helices. ( e ) Positioning of TMDs 1 and 2 of PR directly in front of the lateral gate of SecY. ( f ) Isolated electron density assigned to the TMDs from PR (up) displays high similarity to the corresponding domains in the NMR structure (down) [18] . Full size image For a molecular interpretation of the SecY density, we rigidly fitted a homology model of E. coli SecY based on a SecYEG crystal structure bound to SecA from Aquifex aeolicus [6] . The model was positioned on the large ribosomal subunit via the previously observed and well-resolved contacts of the cytosolic loops 8/9 and 6/7 of SecY ( Fig. 3d ) [7] , [23] , [26] . The TMDs of SecY were then manually adjusted by small shifts into the electron density using COOT [27] . The C-terminal half of SecY as a whole entity fitted remarkably well with only minor changes. The area around helices 1, 4 and 5 of the N-terminal half of SecY was slightly poorly resolved, possibly due to the absence of SecG. The latter is known to be only loosely bound to SecYE [28] and was apparently (at least partially) lost during purification. Helices 2b and 3 of SecY, however, are clearly resolved and could be unambiguously assigned ( Fig. 3d ). In addition, the position of the N-terminal two TMDs of SecE is in agreement with two-dimensional crystal structures of SecYEG [29] and a structure of the SecY-complex in a nanodisc [7] . Moreover, we observe the same overall positioning as well as the same contacts between SecYE and the large ribosomal subunit when compared with the SecYE complex in the membrane environment [7] , indicating that the behaviour of detergent solubilized ribosome-bound SecYE is very similar to that in the lipid bilayer. The estimated local resolution [30] of the SecYE electron density is between 7 and 10 Å, and that of the detergent micelle that surrounds SecYE ≥10 Å ( Supplementary Fig. 3 ). The overall conformation of our SecY model is distinct from that of the template structure (cross-correlation coefficient (c.c.c.)=0.88). It is most similar to the ‘pre-open’ state ( Fig. 4e ) observed by X-ray crystallography [4] (2zjs, c.c.c.=0.90) and, hence, an intermediate between the ‘closed’ ( Fig. 4d ) state [3] (1rhz, c.c.c.=0.83) and the ‘opened’ ( Fig. 4f ) state [5] (3mp7, c.c.c.=0.78; see also Supplementary Fig. 4 ). The plug domain formed by helix 2a of SecY remains essentially the same as observed in the SecA-bound SecYEG structure. 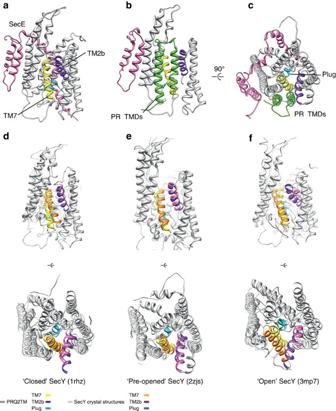Figure 4: Molecular model of the SecYE complex during membrane protein biogenesis. (a) Front view of the lateral gate region of SecY, showing a rather closed conformation of the lateral gate, similar to the ‘pre-activated’ state4. Front view (b) and top view (c) of SecYE inserting the nascent chain PR2Q into the membrane. The nascent chain could not be traced inside the channel. (d–f) Comparison of the tightly coupled PR2Q-SecY with the ‘closed’, ‘pre-opened’ and ‘opened’ SecY crystal structures, respectively. Figure 4: Molecular model of the SecYE complex during membrane protein biogenesis. ( a ) Front view of the lateral gate region of SecY, showing a rather closed conformation of the lateral gate, similar to the ‘pre-activated’ state [4] . Front view ( b ) and top view ( c ) of SecYE inserting the nascent chain PR2Q into the membrane. The nascent chain could not be traced inside the channel. ( d – f ) Comparison of the tightly coupled PR2Q-SecY with the ‘closed’, ‘pre-opened’ and ‘opened’ SecY crystal structures, respectively. Full size image The lateral gate of SecY is more open when compared with a recently published cryo-EM based model of E. coli SecY reconstituted with non-translating ribosomes [31] , but less open when compared with the models of a crosslinked RNC-SecY complex engaging a signal sequence [31] , a RNC-Sec61 (ref. 8 ) complex caught in the moment of inserting a hydrophobic transmembrane segment, as well as a model of SecY engaging a signal anchor determined in the membrane environment [7] . However, the overall conformation of SecY is very similar to the structure of Sec61 translocating a hydrophilic substrate [8] ( Supplementary Figs 4 and 5 ). Crucially, after building the SecYE model, two rod-like densities on the ‘front’ side of SecY remained unaccounted for. We assigned these densities to the first two TMDs of PR that have just left the SecY-complex ( Fig. 3b,c,e,f ). Their position is consistent with the limited length of C-terminal linker between the second PR TMDs and the P-site tRNA, as well as the proximity of the proposed lateral gate of SecY between helices 2b and 7 that may have been used for membrane insertion. Moreover, the unaccounted density strongly resembled the structure of PR TMDs 1 and 2 as obtained by NMR ( Fig. 3f ). The molecular model of PR TMDs 1 and 2 could indeed be fitted as a single rigid body ( Figs 3e and 5a ). Although we cannot draw any conclusions about the path of the two TMDs leading to this position, it is tempting to speculate that the TMDs left the PCC via the proposed lateral gate of SecY. The position of the first two TMDs of PR directly in front of the lateral gate may correspond to the previously proposed secondary binding site(s) for nascent TMDs at the periphery of the Sec-complex [32] . One of two TMDs of PR2Q is in a similar position relative to SecY as a signal anchor [7] or a signal sequence [31] ( Supplementary Fig. 5 ), indicating that signal sequences and TMDs from monotopic as well as polytopic IMPs may enter the lipid bilayer via the same pathway. 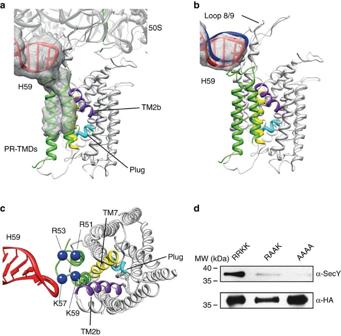Figure 5: Electrostatic interactions between a nascent membrane protein and ribosomal RNA. (a) Continuous electron density reveals a contact between ribosomal RNA helix 59 and the cytoplasmic loop 1/2 of nascent PR2Q. (b) rRNA helix 59 (red) moves towards the membrane region, relative to its canonical position (blue). (c) Top view of the molecular model of helix 59 interacting with the nascent membrane protein. Positively charged residues in loop 1/2 of PR are displayed as blue spheres. (d) Mutation of the positively charged amino acids in loop 1/2 of PR to alanines converts the tightly coupled RNC-SecY complex into a loosely coupled complex (RRKK: wt, RAAK: R53A/K57/A, AAAA: R51A/R53A/K57A/K59A). RNC-SecY complexes were purifiedviaan N-terminal Twin-Strep affinity tag on the nascent chain. Figure 5: Electrostatic interactions between a nascent membrane protein and ribosomal RNA. ( a ) Continuous electron density reveals a contact between ribosomal RNA helix 59 and the cytoplasmic loop 1/2 of nascent PR2Q. ( b ) rRNA helix 59 (red) moves towards the membrane region, relative to its canonical position (blue). ( c ) Top view of the molecular model of helix 59 interacting with the nascent membrane protein. Positively charged residues in loop 1/2 of PR are displayed as blue spheres. ( d ) Mutation of the positively charged amino acids in loop 1/2 of PR to alanines converts the tightly coupled RNC-SecY complex into a loosely coupled complex (RRKK: wt, RAAK: R53A/K57/A, AAAA: R51A/R53A/K57A/K59A). RNC-SecY complexes were purified via an N-terminal Twin-Strep affinity tag on the nascent chain. Full size image Unlike the strong electron density that we observed for PR2Q inside the ribosomal exit tunnel and outside the SecY complex, we did not observe clear density for the FtsQ-derived hydrophilic stretch and therefore we omitted this from our model. Although we cannot formally exclude alternative pathways, we argue that this stretch is most likely retained within the central constriction of SecY for the following reasons: (i) the physicochemical properties of this stretch determine whether or not SecY remains tightly bound to RNCs ( Fig. 2 ); (ii) cysteine residues within a similarly positioned hydrophilic stretch of RNCs have previously been crosslinked to the central constriction of SecY [33] ; and (iii) in a recently published cryo-EM study of Sec61α in a similar conformation as SecY presented here ( Supplementary Fig. 4 ) it was shown that an unstructured stretch of amino acids is able to pass through the central constriction [8] . Structures of SecY/Sec61 complexes with nascent IMPs at higher resolution are eagerly awaited to unambiguously resolve the path of this crucial region of the substrate. Interaction of the nascent IMP with rRNA helix 59 Interestingly, our molecular model of the RNC-SecYE complex shows a direct contact of PR and rRNA helix 59 (H59) of the large ribosomal subunit via the short positively charged loop region that connects TMD 1 and TMD 2 on the cytoplasmic side ( Fig. 5a,c ). Notably, compared with its canonical position [14] , and compared with the structure of SecY in a membrane environment [7] , we observed H59 in a position shifted towards the membrane region ( Fig. 5b ). While Frauenfeld et al. [7] observed a contact of H59 with the lipids in the nanodisc, a direct contact between the nascent IMP and H59 was not observed. Therefore, we tested whether the positively charged residues in between the two TMDs of PR contribute to tight SecY binding. Importantly, mutation of either two or four of these residues to alanine greatly diminished the amount of SecY that was co-purified with the PRQ RNCs ( Fig. 5d and Supplementary Fig. 6 ), indicating a crucial role in stabilizing the ribosome-SecY interaction. Thus, we suggest that a third requirement for tight coupling of the SecY-complex to the ribosome is an electrostatic interaction between the negatively charged rRNA of H59 and positively charged residues in a cytoplasmic domain of the nascent IMP. Taken together, we have presented the first structural snapshot of a nascent polytopic membrane protein during SecY-mediated membrane insertion. The possibility of the ribosome-SecY interaction to alternate between a tightly coupled and a loosely coupled mode may be required for efficient membrane integration of TMDs on one hand, and to allow access of the motor protein SecA for translocation of large extracellular domains on the other hand [34] as it was shown that SecA and SecY cannot bind to the ribosome at the same time [35] . Our structure supports the idea that TMDs of polytopic IMPs indeed may insert into the lipid bilayer by leaving the translocon via the lateral gate, as proposed based on the SecY crystal structure [3] , cryo-EM studies [7] , [31] and crosslinking studies with secretory substrates [36] . The position of the first two TMDs of PR directly in front of the lateral gate most likely corresponds to the previously proposed secondary binding site(s) for nascent TMDs at the periphery of Sec61 (ref. 32 ). More recent crosslinking studies have indicated that the bacterial membrane protein insertase YidC occupies the lateral gate region of SecY [10] , yet we could not identify significant amounts of YidC in our purified RNC-SecY complexes of FtsQ or CyoA ( Supplementary Fig. 7 ). Hence, the interplay between SecY and YidC as well as the motor protein SecA in membrane protein biogenesis remains subject to future studies. Finally, our studies provide a strong hint that the ribosome may be physically involved in determining the topology of IMPs according to the positive inside rule [37] . Although previous studies have pointed at roles for SecY/Sec61 (refs 11 , 12 ), lipids [13] and the transmembrane electrical potential [38] , (although the latter has been contradicted [39] ), a direct role for the ribosome was thus far not implied. An electrostatic interaction between the negatively charged ribosomal RNA helix 59 and nascent IMPs suggests an attractive molecular mechanism for retaining positively charged loop regions on the cytoplasmic side of the membrane during integration into the lipid phase. Support for such a mechanism is provided by the observation that positively charged residues can indeed arrest the movement of nascent proteins through the PCC in a salt-sensitive manner [40] . Our findings thus provide a starting point for designing experiments that address this potential mechanism in more detail. Bacterial strains All RNCs and ribosome nascent chain—SecY complexes were expressed in E. coli KC6 Δ smpB Δ ssrA [15] . Plasmid amplification was carried out in E. coli DH5α cells. Summary of plasmids All RNC constructs were prepared using standard molecular cloning techniques and cloned in the pBAD vector (Invitrogen) using the NcoI and HindIII restriction sites, resulting in an additional glycine after the initiator methionine. DNA primers used for cloning are summarized in detail in Supplementary Table 1 . There is a PstI site between the signal sequence of PR and the Twin-Strep tag, and an ApaI site between the HA tag and the TnaC stalling sequence. SecY was C-terminally tagged with a His 8 -tag and co-expressed with SecE and SecG from the RSFDuet vector (Novagen). Purification of RNCs E. coli KC6 Δ smpB Δ ssrA carrying the plasmid encoding for the respective RNC construct were grown at 37 °C in Lysogeny broth medium to an OD 600 of 0.5. Expression of the nascent chain was induced for 1 h by adding 0.2% arabinose. Cells were harvested and resuspended in buffer A (20 mM Tris pH 7.5, 150 mM NH 4 Cl, 10 mM MgCl 2 1 mM tryptophan, 250 μg ml −1 chloramphenicol and 0.1% EDTA-free complete proteinase inhibitors (Roche Applied Science). Cells were lysed by passing two times through a microfluidizer (M-110L, Microfluidics) and debris were removed by centrifugation for 20 min at 30,000 × g in a SS34-rotor (Sorvall). The cleared lysate was centrifuged for 1 h at 125,000 × g in a Ti45 rotor (Beckman), the resulting crude membrane pellet was resuspended in a small volume of buffer A and then equally divided over several five-step sucrose density gradients consisting of 0.5 ml 55, 50, 45, 40 and 35% sucrose in buffer A in a TLA110 (Beckman) tube. After spinning for 30 min at 417,000 × g, the brownish layer of inner membranes was taken out from the lower third of the tube and subsequently solubilized in buffer A+1% DDM (n-Dodecyl β-D-maltopyranoside). Ribosomes carrying the nascent chain were separated by affinity chromatography using StrepTactin Beads (IBA) or Talon (Clonetech). Talon beads were additionally pre-incubated with 10 μg ml −1 E. coli tRNAs to minimize unspecific binding of ribosomes. After incubating for 1 h at 4 °C, the beads were washed with at least 10 column volumes of buffer B (20 mM Tris pH 7.5 150 mM NH 4 Cl, 10 mM MgCl 2 250 mM sucrose, 0.1% DDM). RNCs were eluted in buffer B+2.5 mM desthiobiotin or 150 mM imidazole and loaded on a linear sucrose gradient 10–40% sucrose in buffer B. After spinning for 3 h at 202,000 × g in a SW40 rotor (Beckman), the 70S peak was collected and diluted three times with buffer B. RNCs were finally concentrated by spinning for 4 h at 117,000 × g in a Ti70 rotor (Beckman) and resuspended in an appropriate volume of buffer B. RNCs were flash frozen in liquid N 2 and stored at −80 °C RNC-SecY complex purification for cryo-EM data collection E. coli KC6 Δ smpB Δ ssrA were transformed with a plasmid encoding for the respective nascent chain in pBAD and SecY(His)EG and grown in Lysogeny broth at 37 °C to an OD 600 of 0.5. The nascent chain was induced for 1 h by adding 0.2% arabinose. Expression of SecY(His)EG was not induced. Inner membranes were isolated and solubilized as described above for the purification of RNCs. SecY-RNC complexes were purified on Talon beads (Clonetech), pre-incubated in buffer B+20 mM imidazole and 10 μg ml −1 E. coli tRNAs to minimize unspecific binding of ribosomes. After washing the beads with 50 column volumes buffer B+20 mM imidazole, SecY-RNC complexes were eluted in buffer B+250 mM imidazole. Isolation of monosomal complexes over a linear sucrose gradient and final concentration was performed as described above. Western blot analysis SDS gels were blotted on PVDF membrane (Millipore) using a semidry electro blotter (Peqlab). Working dilutions of all antibodies and catalogue numbers of purchased antibodies are listed in Supplementary Table 2 . Full scans of the western blots are shown in Supplementary Fig. 8 . Cryo-EM and image processing The freshly prepared PR2Q-RNC-SecYEG complex was applied to 2 nm pre-coated Quantifoil R3/3 holey carbon supported grids and vitrified using a Vitrobot Mark IV (FEI Company). Cryo-EM data were collected on a Titan Krios TEM (FEI Company) under low-dose conditions (~20 e − /Å 2 ) at 200 keV and a magnification of × 148,721 at the plane of the CCD on a TemCam-F416 CMOS camera (TVIPS GmbH, 4,096 × 4,096 pixel, 15.6 μm pixel, 1 s per full frame) resulting in a pixel size of 1.049 Å and a nominal defocus between −1 μm and −3.5 μm. Data were processed using the SPIDER [41] software package. The CTF was determined using the TF ED command from SPIDER and particles were selected automatically using the program SIGNATURE [42] . After initial selection of particles, a second selection for particles against contaminations, noise, ice, carbon edges, and so on was performed using a newly developed machine learning algorithm, MAPPOS [43] . The data set of 567,343 particles was first sorted for the presence of only P-site tRNA (267,311 with P-site tRNA) and subsequently sorted for the presence of SecYE at the ribosomal tunnel exit resulting in a volume reconstructed of 135,010 particles, that could be refined to 7.5 Å (FSC 0.5). Since the density for SecYE still displayed heterogeneity, possibly due to the presence of nascent chain only, signal recognition particle or a cytosolic chaperone bound to the nascent chain, the data were further sorted focusing on the SecY region resulting in a stable subpopulation of 47,471 particles that could be refined to 7.3 Å (FSC 0.5). Model building for the E. coli PR2Q-RNC-SecYE complex For the generation of homology models, the programs HHPRED [44] and MODELLER [45] were used. For building a homology model from E. coli SecY, the model of A. aeolicus SecY in complex with Bacillus subtilis SecA [6] was used as a reference and modelled in the electron density using COOT [27] and UCSF Chimera [46] . The nascent chain was modelled using an NMR structure of PR [18] for the PR part of the hybrid nascent chain. The ribosomal model was based on a TnaC-stalled ribosome [14] . Accession codes: The Cryo-EM density map has been deposited in the EMDB under accession code EMDB-2446. How to cite this article: Bischoff, L. et al. Visualization of a polytopic membrane protein during SecY-mediated membrane insertion. Nat. Commun. 5:4103 doi: 10.1038/ncomms5103 (2014).